Climate change patterns in Amazonia and biodiversity Precise characterization of hydroclimate variability in Amazonia on various timescales is critical to understanding the link between climate change and biodiversity. Here we present absolute-dated speleothem oxygen isotope records that characterize hydroclimate variation in western and eastern Amazonia over the past 250 and 20 ka, respectively. Although our records demonstrate the coherent millennial-scale precipitation variability across tropical–subtropical South America, the orbital-scale precipitation variability between western and eastern Amazonia exhibits a quasi-dipole pattern. During the last glacial period, our records imply a modest increase in precipitation amount in western Amazonia but a significant drying in eastern Amazonia, suggesting that higher biodiversity in western Amazonia, contrary to ‘Refugia Hypothesis’, is maintained under relatively stable climatic conditions. In contrast, the glacial–interglacial climatic perturbations might have been instances of loss rather than gain in biodiversity in eastern Amazonia, where forests may have been more susceptible to fragmentation in response to larger swings in hydroclimate. Amazonia is home to the richest terrestrial biodiversity on Earth. It also serves as a massive source of heat and moisture in the tropics and has a crucial role in the global climate system, having impacts on precipitation variations across both hemispheres [1] . Although the evolutionary history and spatial patterns of Amazon biodiversity are now essentially well established [2] , the long-term climate variability and its potential influence on the biodiversity remain poorly understood. Precise characterization of hydroclimate variability in Amazonia on a wide range of timescales is of vital importance to understanding the possible link between climate change and biodiversity, and a necessary step towards an assessment of the spatial–temporal patterns of tropical forest response to potential future climate change in South America. Despite a growing body of paleoclimate data from the region ( Fig. 1 ; Supplementary Fig. S1 ), patterns of hydrologic variation in Amazonia, particularly in the biodiversity core area of western Amazonia, are poorly documented beyond the Holocene [3] . Thus, it remains unclear whether or how orbital-to-millennial-scale climate variability manifested itself in Amazonia and how it was linked to adjacent regions. 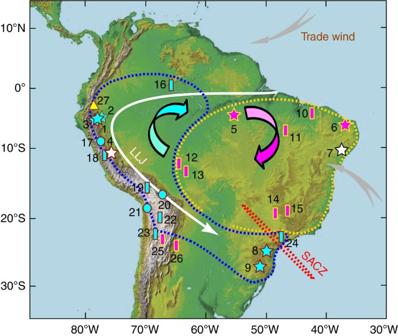Figure 1: Location of climate records from South America and current regional climate patterns. Also shown are some major components of the SAM, including South Atlantic convergence zone (SACZ, red dashed lines) and low-level jet (LLJ, white arrow) (adapted from ref.19). The blue/orange circles indicate the SAPD, consistent with modern precipitation pattern26and simulation results7,21. Stars indicate caves: 1. ELC, 2. NAR, 3. Cueva del Tigre Perdido, 4. Pacupahuain. 5. Paraíso, 6. Rio Grande do Norte, 7. Toca da Boa Vista, 8. Santana and 9. Botuverá. Rectangles and circles (10–27) show lake and ice core records, respectively. Light blue and purple symbols indicate wet and dry LGM, respectively25, and white show wet condition during Heinrich events (Supplementary Fig. S1). Yellow triangle depicts the Surucucho pollen record32that indicates little change in forest composition throughout the Holocene. Two wide arrows show the east–west zonal overturning circulation during strong SAM times with ascending and descending motions over western and eastern Amazonia, respectively21. Figure 1: Location of climate records from South America and current regional climate patterns. Also shown are some major components of the SAM, including South Atlantic convergence zone (SACZ, red dashed lines) and low-level jet (LLJ, white arrow) (adapted from ref. 19 ). The blue/orange circles indicate the SAPD, consistent with modern precipitation pattern [26] and simulation results [7] , [21] . Stars indicate caves: 1. ELC, 2. NAR, 3. Cueva del Tigre Perdido, 4. Pacupahuain. 5. Paraíso, 6. Rio Grande do Norte, 7. Toca da Boa Vista, 8. Santana and 9. Botuverá. Rectangles and circles (10–27) show lake and ice core records, respectively. Light blue and purple symbols indicate wet and dry LGM, respectively [25] , and white show wet condition during Heinrich events ( Supplementary Fig. S1 ). Yellow triangle depicts the Surucucho pollen record [32] that indicates little change in forest composition throughout the Holocene. Two wide arrows show the east–west zonal overturning circulation during strong SAM times with ascending and descending motions over western and eastern Amazonia, respectively [21] . Full size image Here we present new absolute-dated speleothem oxygen isotope records to establish the spatio-temporal patterns of hydroclimate variation over the past 250 and 20 ka in western and eastern Amazonia, respectively. Together with existing climate proxy data, we unveil the dominant patterns of precipitation variability on orbital–millennial timescales across tropical–subtropical South America and in turn to probe possible linkages between climate change and biodiversity. Cave location We collected a suite of stalagmites from El Condor (ELC) (5°56′S, 77°18′W, 860 m a.s.l), Cueva del Diamante (NAR) (5°44′S, 77°30′W, 960 m a.s.l.) caves, which are located within the core biodiversity region on the eastern flank of the Andes in northern Peru ( Fig. 1 ). The mean annual precipitation in this region is ca. 1,500 mm, 80% of which falls in austral summer when the South American monsoon (SAM) circulation transports tropical Atlantic moisture, which is largely recycled over the Amazon Basin, westward towards the Andes. The warm and humid air masses are deflected southward by the Andes, fuelling the Andean low-level jet, transporting moisture towards southeastern South America ( Fig. 1 ). During the austral winter, the SAM completely disappears and gives way to a strong mid- and upper-tropospheric subtropical jet stream [4] . Speleothem δ 18 O records Our western Amazon speleothem δ 18 O records cover most portion of the past 250 ka ( Fig. 2 ; Supplementary Figs S2–S4 ). Modern hydrological data and various model simulations suggest that precipitation amount and degree of upstream rainfall/transpiration are two primary factors that influence the δ 18 O of precipitation at our sites. The long east-to-west transport of the moisture from the tropical Atlantic across the Amazon Basin towards the cave sites in the tropical Andes leads to a progressively lower δ 18 O value of precipitation caused by rainout upstream, namely the ‘continental effect’ [5] , [6] , [7] ( Supplementary Figs S5 and S6 ). However, this effect is smaller than expected from observed intense rainout along the trajectory, because the strong water recycling over the Amazon Basin recharges the atmosphere with relatively 18 O-enriched water vapor [8] , [9] , [10] . Moreover, the δ 18 O of precipitation has been shown to be inversely correlated with the amount of rainfall, a relationship dubbed as the ‘amount effect’, with a slope between −0.4 and −0.8‰ per 100 mm increase in the mean annual precipitation [11] . In contrast, the ‘temperature effect’ on the δ 18 O of modern summer precipitation in tropical South America is insignificant [3] , [6] , [11] , [12] , [13] . We, thus, interpret the δ 18 O variations in our record, particularly the relatively large amplitude changes on orbital timescale upon which we focus here, to primarily reflect variations in SAM precipitation amount and degree of upstream rainfall/transpiration [14] . 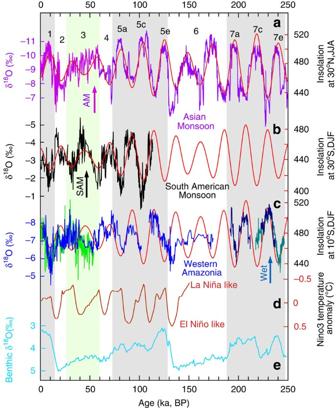Figure 2: Speleothem δ18O records from western Amazonia in comparison with other climate records. (a) AM records (purple: Hulu-Dongge caves; dark purple: Sanbao cave)15,45and boreal summer (JJA) insolation at 30°N (ref.47). (b) Southern Brazil records (Botuverá cave)18and ASI (DJF) at 30°S(ref.47). (c) Western Amazon records and ASI (DJF) at 10°S(ref.47). (d) Niño3 temperature anomalies estimated with the Zebiak and Cane model48depict the variability of orbital ENSO mean state. (e) The stacked benthic δ18O record49. Numbers at the top indicate MISs. Arrows depict an increase of the AM and the SAM. The typical SAM record from southern Brazil follows ASI and thus displays a broad anti-phase relationship to the AM. In contrast, while the record from western Amazonia tracks ASI during relatively warm periods (MIS 1, 5 and 7) when sea level was higher, it shows an apparently anti-phase relationship to some extent to ASI during relatively cold periods (MIS 2–4 and 6) when sea level was lower (seeSupplementary Fig. S11for more details). To first order, the ENSO counterbalances and reinforces orbital SAM variations in western Amazonia and eastern Amazonia-northeastern-southern Brazil, respectively (seeSupplementary Figs S9 and S10for details). Figure 2: Speleothem δ 18 O records from western Amazonia in comparison with other climate records. ( a ) AM records (purple: Hulu-Dongge caves; dark purple: Sanbao cave) [15] , [45] and boreal summer (JJA) insolation at 30°N (ref. 47 ). ( b ) Southern Brazil records (Botuverá cave) [18] and ASI (DJF) at 30°S(ref. 47 ). ( c ) Western Amazon records and ASI (DJF) at 10°S(ref. 47 ). ( d ) Niño3 temperature anomalies estimated with the Zebiak and Cane model [48] depict the variability of orbital ENSO mean state. ( e ) The stacked benthic δ 18 O record [49] . Numbers at the top indicate MISs. Arrows depict an increase of the AM and the SAM. The typical SAM record from southern Brazil follows ASI and thus displays a broad anti-phase relationship to the AM. In contrast, while the record from western Amazonia tracks ASI during relatively warm periods (MIS 1, 5 and 7) when sea level was higher, it shows an apparently anti-phase relationship to some extent to ASI during relatively cold periods (MIS 2–4 and 6) when sea level was lower (see Supplementary Fig. S11 for more details). To first order, the ENSO counterbalances and reinforces orbital SAM variations in western Amazonia and eastern Amazonia-northeastern-southern Brazil, respectively (see Supplementary Figs S9 and S10 for details). Full size image Millennial-scale variability Our western Amazon δ 18 O profiles are characterized by numerous millennial-scale abrupt shifts with amplitude of ~1.5‰ ( Figs 3 and 4 ; Supplementary Figs S7 and S8 ). These events correspond with the Younger Dryas (YD), Dansgaard-Oeschger (D/O) and Heinrich (H) events, and are, within dating error, anti-phased with their Northern hemisphere (NH) counterparts such as changes in Asian monsoon (AM) [15] , Greenland temperature [16] and the Cariaco Basin records [17] , and in-phase with speleothem records from southern [18] , [19] and northeastern Brazil [20] , [21] and high altitude central Peruvian Andes [14] , and the Lake Titicaca record [22] ( Supplementary Figs S7 and S8 ). The interhemispheric anti-phased nature of these events supports the notion that the H-YD (low δ 18 O excursions) and D/O (high δ 18 O excursions) events manifest in South America as wet and dry episodes, respectively. The abrupt increase in monsoon rainfall during the H-YD events is likely related to a southward shift in the mean position of the ITCZ, a strengthening of the asymmetry in Hadley circulation in response to an inter-hemispheric gradient of sea surface temperature and to some extent a possible influence from Antarctic climate changes [14] , [19] , [20] . 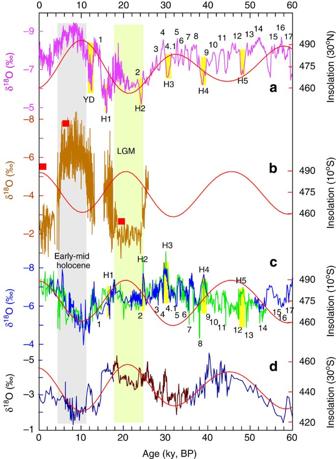Figure 3: Comparison among speleothem δ18O records over the past 60 ka. (a) AM records (Hulu-Dongge)15,45and boreal summer (JJA) insolation47. (b) Rio Grande do Norte record, northeastern Brazil (brown)21and the typical LGM, mid Holocene and modern δ18O values (red squares) obtained from Paraíso cave, eastern Amazonia. Red curve is ASI (DJF)47. (c) Western Amazon records (blue-the NAR record, green-the ELC record). Red curve shows ASI (DJF)47. (d) Botuverá cave δ18O records, southern Brazil18,19and ASI (DJF)47. Two large vertical bars depict the early-mid Holocene and the LGM, respectively. Yellow bars show H events. Numbers indicate Greenland interstadials. The striking anti-phase relationship over the last precession cycle is apparent between eastern Amazonia-northeastern Brazil and western Amazonia-southern Brazil (Fig. 1). Despite the difference on orbital scale (Fig. 2), the millennial events show a coherent pattern in tropical–subtropical South America, which is anti-phased with their AM counterparts (Fig. 4). Figure 3: Comparison among speleothem δ 18 O records over the past 60 ka. ( a ) AM records (Hulu-Dongge) [15] , [45] and boreal summer (JJA) insolation [47] . ( b ) Rio Grande do Norte record, northeastern Brazil (brown) [21] and the typical LGM, mid Holocene and modern δ 18 O values (red squares) obtained from Paraíso cave, eastern Amazonia. Red curve is ASI (DJF) [47] . ( c ) Western Amazon records (blue-the NAR record, green-the ELC record). Red curve shows ASI (DJF) [47] . ( d ) Botuverá cave δ 18 O records, southern Brazil [18] , [19] and ASI (DJF) [47] . Two large vertical bars depict the early-mid Holocene and the LGM, respectively. Yellow bars show H events. Numbers indicate Greenland interstadials. The striking anti-phase relationship over the last precession cycle is apparent between eastern Amazonia-northeastern Brazil and western Amazonia-southern Brazil ( Fig. 1 ). Despite the difference on orbital scale ( Fig. 2 ), the millennial events show a coherent pattern in tropical–subtropical South America, which is anti-phased with their AM counterparts ( Fig. 4 ). 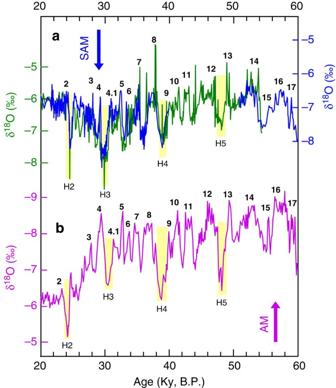Figure 4: Precise anti-correlation between the millennial variability of the AM and the SAM. (a) Northern Peru δ18O records from NAR (blue) and ELC (green) caves. (b) The AM δ18O record from Hulu cave15. The δ18O scale is reversed for the Hulu record (increasing down) as compared with Peruvian records (increasing up). The vertical bars depict H2 to H5. Numbers indicate Greenland interstadials. It is now evident that the SAM is precisely anti-phased with the AM in millennial variability, including YD, D/O H events. Full size image Figure 4: Precise anti-correlation between the millennial variability of the AM and the SAM. ( a ) Northern Peru δ 18 O records from NAR (blue) and ELC (green) caves. ( b ) The AM δ 18 O record from Hulu cave [15] . The δ 18 O scale is reversed for the Hulu record (increasing down) as compared with Peruvian records (increasing up). The vertical bars depict H2 to H5. Numbers indicate Greenland interstadials. It is now evident that the SAM is precisely anti-phased with the AM in millennial variability, including YD, D/O H events. Full size image Orbital timescales variability Although the millennial-scale precipitation variability across tropical South America has a largely coherent pattern; the spatial structure of precipitation is complex on orbital timescales. This is evident from the comparison of existing speleothem δ 18 O records from southern and northeastern Brazil with our speleothem records from western (Peruvian caves) and eastern (Paraíso cave) Amazonia. The western Amazonia and southern Brazil δ 18 O variations are broadly in-phase to first order, reflecting changes in the SAM intensity [7] , [11] , [18] resulting from changes in austral summer insolation (ASI) associated with the precession cycle [18] ( Fig. 2 ). In addition, they are anti-phased with their NH counterpart, the AM [15] , [23] , supporting the notion that increased summer solar radiation is the most effective factor strengthening tropical–subtropical monsoons [23] , [24] . The western Amazonia and southern Brazil speleothem records are, however, out of phase with speleothem records from northeastern Brazil [21] and eastern Amazonia ( Fig. 3 ). A notable feature of the latter records is a significantly larger δ 18 O variance over the last precession cycle (~5–6‰) ( Fig. 3 ). South American precipitation dipole We define the observed east–west dipole-like pattern of precipitation changes during the last precession cycle as the South American precipitation dipole (SAPD) ( Figs 1 and 3 ). The precession-scale SAPD is consistent with other paleoclimate reconstructions during the last glacial maximum (LGM) in South America [25] ( Fig. 1 ; Supplementary Fig. S1 ) and is akin to the precipitation amount and δ 18 O dipole patterns, as observed in instrumental data and modelling simulations [7] , [21] , [26] . On the precession scale, the SAPD may be dynamically linked to the SAM variability as follows. When high ASI intensifies the SAM, strong convective activity and upward motion result in enhanced condensational heating over the western Amazon Basin, which in turn intensifies the upper-tropospheric Nordeste low and results in large-scale subsidence and aridity over eastern equatorial South America [21] , [27] . In addition, the SAPD phenomenon may contribute to the observed global atmospheric δ 18 O and CH 4 changes that closely follow NH AM variations on precession scale [15] , [28] . As the precipitation signal over eastern tropical South America essentially follows NH insolation, the overall influence of the Southern Hemisphere precession signal on global atmospheric δ 18 O and CH 4 concentrations is likely significantly reduced. El Niño–Southern oscillation influence In tropical South America, however, El Niño–Southern oscillation (ENSO) can also have a substantial effect on precipitation. Instrumental observations suggest that the El Niño (La Niña) episodes are generally associated with below (above) average precipitation and higher (lower) δ 18 O in western-eastern Amazonia and northeastern Brazil (southern Brazil) [11] , [29] , [30] ( Supplementary Fig. S9 ). Given the different ENSO–SAPD spatial patterns, it is thus conceivable that precipitation changes associated with long-term changes in ENSO mean state may counterbalance precession-induced precipitation variability in western Amazonia, while reinforcing it in northeastern-southern Brazil and eastern Amazonia ( Supplementary Figs S9 and S10 ). Our δ 18 O records from western Amazonia exhibit fluctuations of ~3‰ that track variations of the ASI at times when the global ice volume was smaller during marine isotope stage (MIS) 1, 5 and 7. In contrast, the δ 18 O variation during times of larger global ice volume is of smaller amplitude (~2‰) on the precession scale. The modulating influence of orbital-scale shifts in ENSO mean state could potentially explain why δ 18 O changes in western (eastern) Amazonia are of smaller (larger) amplitude ( Fig. 2 ). The former, to second order, appears to mimic the ENSO change, rather the ASI ( Supplementary Figs S10 and S11 ). This apparent distinction in the covariance between the δ 18 O and insolation might imply a possible weaker (stronger) ENSO influence under the interglacial (glacial) condition or a stronger and more complex influence from glacial boundary conditions on the precipitation over tropical South America [31] . Speleothem δ 18 O records from northeastern Brazil and eastern Amazonia reveal a large-scale decrease in δ 18 O values (5–6‰) from the LGM to the early-mid Holocene (~10–5 ka BP) ( Fig. 3 ), implying a drastic shift from severely dry to substantially wet conditions in the region where the ‘amount effect’ on precipitation δ 18 O is presumed to be dominant [21] . In contrast, over the same time interval, our western Amazon records indicate a high δ 18 O excursion with smaller amplitude (~2‰) change, which we interpret to reflect a shift from relatively wet to moderately dry conditions ( Fig. 3 ). This is in accordance with lake records that had documented a wetter LGM versus a drier early-mid Holocene in western Amazonia and many Andean sites ( Fig. 1 ). During the early-mid Holocene when the SAM was weak [18] , western Amazon speleothem records are characterized by the highest δ 18 O value of the entire record, likely suggesting driest conditions during the past two glacial–interglacial cycles ( Fig. 2 ). With regard to climate impacts on ecosystems, the degree of severity of the early-mid Holocene dry phase in western Amazonia is an important issue. Recent work based on isotope studies of fluid inclusions in speleothems from the region provides estimates of temperature and rainfall changes during the Holocene [3] . The temperature change was found to be trivial throughout the Holocene but the rainfall amount was reduced by 15–30% below present day as inferred from the modern amount effect on the δ 18 O (−0.4 to −0.8‰ per 100 mm rainfall increase [11] ). The SAM was weak during the early-mid Holocene ( Fig. 3 ), as documented by southern Brazil records [18] . Thus, one may expect a diminution of the moisture from distant source (lower δ 18 O moisture from the Atlantic) in western Amazonia. Meanwhile, a much wetter eastern Amazonia during the early-mid Holocene, inferred by the extremely low δ 18 O, implies that the moisture transported to downstream western Amazonia would be much more depleted due to Rayleigh distillation. This simple mechanism, [14] however, appears insufficient to explain the fact that the δ 18 O of precipitation in western Amazonia became much higher, rather than lower, or absolute rainfall δ 18 O values in both eastern and western Amazonia is essentially the same. As such, a most likely interpretation would be that the dominant moisture transported to western Amazonia is the recycled water vapour through increasing transpiration in eastern Amazonia upstream, as transpiration is typically a non-isotope fractionating process. It is, in turn, likely that hydrological fluctuations in western Amazonia might even be smaller and the estimate of 15–30% rainfall decrease may be an utmost face value, because a portion of the high δ 18 O excursion may also result from a higher δ 18 O moisture source or a lower percentage of 18 O-depleted remote moisture rather than from the amount affect. A supporting line of evidence comes from numerous pollen records within and around the Amazon Basin. In contrast to most pollen records in the region that clearly exhibit vegetation changes during the Holocene, the record nearest to our cave site from Lake Surucucho, Ecuador, indeed shows little change in forest composition throughout the Holocene [32] ( Fig. 1 ), supporting the notion from cave records that the rainfall amount reduce may be relatively small in western Amazonia during its dry phase of the early-mid Holocene. This interpretation is consistent with paleoclimate records and simulations available so far, however, the other mechanism cannot, at this stage, be conclusively excluded. Paleoclimate patterns described above provide a new context for further understanding the tropical South American biodiversity. To first order, hypotheses for the origin of the extremely high Amazon diversity have been based on the dichotomy between environmental stability versus instability as drivers of species accumulation [33] , [34] , [35] . The fundamentally different history of climate evolution in eastern and western Amazonia evidenced here as the SAPD pattern for glacial–interglacial or precession cycles provides an opportunity to contribute to this debate. Our analysis indicates that the climate in eastern Amazonia swung drastically between dry and wet conditions during the termination of the last ice age and, whereas in contrast, conditions in western Amazonia might not have changed as much over the last 250 ka. These climatic patterns may be typical of the Quaternary, as the current South American climatic framework had been established since the pre-Quaternary [2] . These climatic patterns also provide a testable prediction on past biotic interchanges among Amazon, Andean and Atlantic forests [36] , [37] , [38] . The broad similarities in climate history on the glacial–interglacial cycle might be in favour of biotic exchanges along two preferential corridors: one connecting climatically eastern Amazonia with northern Atlantic forests (eastern corridor), and another connecting western Amazonia with southern Atlantic forests (western corridor) ( Supplementary Figs S1 and S12 ). Patterns of distribution of South America birds agree with these predictions ( Supplementary Fig. S13 ). In addition, the pollen records from the predicted corridor areas in northeastern Brazil (eastern corridor) [39] , [40] indicate late Pleistocene forest expansion in a region currently dominated by semi-arid Caatinga vegetation, while in Bolivia (western corridor) two pollen sites show a pattern consistent with a southward increase in forest cover during the last 3,000 years [41] . Both of these independent data sets support the key paleoclimate pattern that we establish here. According to the climate pattern described here, western Amazonia has had a more stable climate, which, combined with richer soils originated from Andean sediments, may be related to the west–east diversity gradient that has been detected for some groups of Amazon organisms, such as trees and mammals [2] . This suggests that a favourable and/or relatively stable climate may be an important factor in driving diversification, either through an increase in speciation rates or a decrease in extinction rates [42] , [43] , or both. Instead, greater climate instability with forest fragmentation during glacial times (the ‘Refugia Hypothesis’ [33] ), a possible scenario in eastern Amazonia, may have been an instance of loss rather than gain in biodiversity. Sample preparation Stalagmites ELC-A and ELC-B are ~57 and 46 cm high and ~7 and 8 cm wide, respectively. Stalagmites NAR-C, D and F are ~120, 52 and 68 cm high and 10–20, 10 and 10 cm wide, respectively. The measured cave temperature and relative humidity in August 2006 are ~22 °C, 92% and 21 °C, 91% for ELC and NAR caves, respectively. All five stalagmites were halved along the growth axis and their surfaces polished. Stable isotope analysis Each subsample for δ 18 O analysis was milled using 0.3-mm carbide dental burrs along the central growth axis. The δ 18 O analyses of samples ELC-A and B were performed with an online automated carbonate preparation system linked to a VG Prism II isotope ratio mass spectrometer at the University of Southern California, whereas samples NAR-C, -D and -F were measured with an online automated carbonate preparation system linked to a Finnigan Delta Plus Advantage at the University of São Paulo. Data were calibrated against standards, NBS-18 and NBS-19, and are reported as δ 18 O (‰) relative to the Vienna Pee Dee Belemnite. Duplicates were analysed every 10–20 samples to check for homogeneity, all of which replicated within 0.12‰. Our western Amazon speleothem δ 18 O records have been constructed from five stalagmites (ELC-A, ELC-B, NAR-C, NAR-D and NAR-F), with an average temporal resolution of ~80 years ( Supplementary Fig. S4 ). 230 Th dating method The chronology is based on 197 230 Th ages. The chemical procedures used to separate U and Th for 230 Th dating are similar to those described in Edwards et al . [44] 230 Th dating of stalagmites was performed at the Minnesota Isotope Laboratory on a multi-collector inductively coupled plasma mass spectrometer (MC-ICPMS, Thermo-Finnigan Neptune). All U and Th isotopes were measured on a MasCom multiplier behind the retarding potential quadrupole in peak-jumping mode. The analytical methods are described in refs 45 and 46 . All dates are in stratigraphic order, with a typical relative 2σ error of better than 1%. The chronology is established using linear interpolation between dates ( Supplementary Table S1 ; Supplementary Figs S2 and S3 ). Three NAR stalagmites grew over the most portion of the past 250 ka and two ELC stalagmites span the last 54 ka. Replication test A high degree of replication between ELC-B and NAR-C δ 18 O profiles from two caves over a 50-ka contemporaneous growth period, 54–4 ka BP (before present, present=1950 AD) ( Figs 3 and 4 ; Supplementary Figs S7 and S8 ), argues against any substantial kinetic effect on δ 18 O values. How to cite this article: Cheng, H. et al . Climate change patterns in Amazonia and biodiversity. Nat. Commun. 4:1411 doi: 10.1038/ncomms2415 (2013).